STV11encodes a sulphotransferase and confers durable resistance to rice stripe virus Rice stripe virus (RSV) causes one of the most serious viral diseases of rice (Oryza sativa L.), but the molecular basis of RSV resistance has remained elusive. Here we show that the resistant allele of rice STV11 ( STV11-R ) encodes a sulfotransferase (OsSOT1) catalysing the conversion of salicylic acid (SA) into sulphonated SA (SSA), whereas the gene product encoded by the susceptible allele STV11-S loses this activity. Sequence analyses suggest that the STV11-R and STV11-S alleles were predifferentiated in different geographic populations of wild rice, Oryza rufipogon , and remained prevalent in cultivated indica and japonica rice varieties, respectively. Introgression of the STV11-R allele into susceptible cultivars or heterologous transfer of STV11-R into tobacco plants confers effective resistance against RSV. Our results shed new insights into plant viral defense mechanisms and suggest effective means of breeding RSV-resistant crops using molecular marker-assisted selection or genetic engineering. Rice (Oryza sativa L.) is a staple food for more than half of the world’s population. Rice stripe virus (RSV), an RNA virus belonging to the genus Tenuivirus and transmitted by small brown planthoppers (SBPH; Laodelphax striatellus Fallen), causes one of the most destructive rice diseases [1] , [2] , [3] . Over 80% of the rice fields in Eastern China ( http://www.hzag.gov.cn/bcjb/200559154000.htm ) and Korea were affected by this disease annually [3] . RSV-infected plants typically display chlorosis, weakness and necrosis in emerging leaves, and as a result their growth is stunted. In severe cases, RSV can cause complete loss of grain yield [3] . Due to the lack of effective remedy for controlling RSV itself, insecticides have been widely used to control its transmitting vector SBPH, which, however, is both costly and harmful to human beings, livestock and the environment. Development of resistant rice cultivars is considered the most economic, effective and environment-friendly measure for controlling this viral disease. The majority of japonica varieties cultivated in East Asia is highly susceptible to RSV. Compared with japonica , a large number of indica cultivars have been shown to be resistant to RSV [1] , [2] , [4] . Although durable RSV resistance has been achieved in some japonica varieties by introgression of resistance genes from indica [4] , such conventional breeding is extremely difficult and time consuming due to the lack of an effective RSV resistance evaluation system and limited knowledge on RSV resistance genes. Despite that five indica -derived major RSV resistance quantitative trait locus (QTLs) ( Stv-bi , qSTV11 IR24 , qSTV11 TQ , qSTV11 KAS and qSTV11 SG ) have been mapped to the long arm of rice chromosome 11 (refs 5 , 6 , 7 , 8 , 9 ), but none of them has been cloned. Thus, the molecular mechanism involved in RSV resistance in rice remains elusive. We previously showed that an Indian landrace Kasalath (KAS) is highly resistant to RSV [8] . A major QTL derived from KAS, qSTV11 KAS (designated STV11-R for resistance to RSV on chromosome 11 in this study), was fine mapped to rice chromosome 11 (ref. 8 ). Here, we report cloning of STV11 and show that STV11 encodes a sulfotransferase, catalysing the conversion of salicylic acid (SA) to sulphonated SA (SSA). Further, we find that two alleles, STV11-R and STV11-S , are prevalent in indica and japonica , respectively, thus explaining the differentiation in RSV resistance between the two subspecies. Our results provide new insights into the molecular mechanisms governing plant-virus interactions. STV11 inhibits RSV replication Koshihikari (Kos) is the most popular japonica variety in Japan and has been widely used in breeding programs due to its popular palatability [10] , but is highly susceptible to RSV [8] . When infested with RSV-carrying SBPH, Kos leaves started to show disease symptoms at about 20 days post infection (d.p.i. ), whereas KK34, a near isogenic line carrying STV11 from KAS in the background of Kos [8] , did not display any visible symptoms during the whole infection process ( Fig. 1a–c ). Evaluation of SBPH resistance showed that both KK34 and Kos were similarly susceptible to SBPH ( Fig. 1d and Supplementary Fig. 1a,b ). Thus, RSV resistance conferred by STV11 is independent of SBPH resistance. 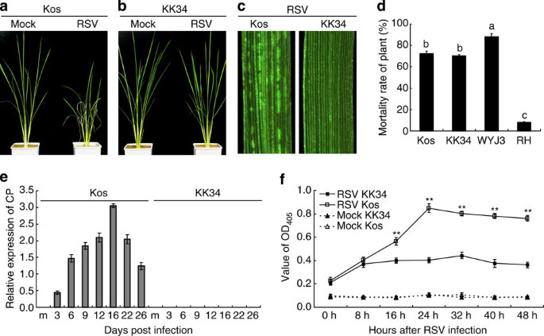Figure 1: Characterization of RSV resistance in KK34. (a,b) Phenotypes of Kos and KK34 plants at 45 d.p.i. with non-virulent (mock) or RSV-carrying SBPH. (c) Representative images of Kos and KK34 leaves. (d) KK34 has similar SBPH susceptibility to Kos. WYJ3 (Wuyujing 3) and RH (Rathu Heenati) were used as the SBHP-susceptible and -resistant control, respectively. Error bars indicate s.e.m. (n=3), different letters at the top of each column indicate significant differences atP<0.01 (n=3) by the Student’st-test. (e) RT–PCR assay showing accumulation of the RSV coat protein mRNA in whole seedling plant without roots of Kos and KK34 following RSV infection. m, mock seedlings were sampled 3 d.p.i. with RSV-free SBPH. The mean±s.e.m. was obtained from three technical repeats and three biological repeats. (f) ELISA assay showing replication of RSV in Kos and KK34 protoplasts. Mock, the protoplasts treated the PBS buffer. Error bars indicate s.e.m. (n=3), **indicates significant differences between Kos and KK34 inoculated with RSV at same time point atP<0.01 (n=3) by the Student’st-test. Figure 1: Characterization of RSV resistance in KK34. ( a , b ) Phenotypes of Kos and KK34 plants at 45 d.p.i. with non-virulent (mock) or RSV-carrying SBPH. ( c ) Representative images of Kos and KK34 leaves. ( d ) KK34 has similar SBPH susceptibility to Kos. WYJ3 (Wuyujing 3) and RH (Rathu Heenati) were used as the SBHP-susceptible and -resistant control, respectively. Error bars indicate s.e.m. ( n =3), different letters at the top of each column indicate significant differences at P <0.01 ( n =3) by the Student’s t -test. ( e ) RT–PCR assay showing accumulation of the RSV coat protein mRNA in whole seedling plant without roots of Kos and KK34 following RSV infection. m, mock seedlings were sampled 3 d.p.i. with RSV-free SBPH. The mean±s.e.m. was obtained from three technical repeats and three biological repeats. ( f ) ELISA assay showing replication of RSV in Kos and KK34 protoplasts. Mock, the protoplasts treated the PBS buffer. Error bars indicate s.e.m. ( n =3), **indicates significant differences between Kos and KK34 inoculated with RSV at same time point at P <0.01 ( n =3) by the Student’s t -test. Full size image To test whether RSV resistance influences viral replication, the transcripts of the RSV coat protein (CP) were measured. The results showed that the transcripts of CP reached a maximum at 16 d.p.i. in Kos but could not be detected in KK34 throughout the course of RSV infection ( Fig. 1e ). To further validate this, we introduced purified RSV ribonucleoprotein particles into rice protoplasts by the polyethylene glycol method. Significantly higher rate of RSV replication was found in Kos than that in KK34 ( Fig. 1f ). These results together suggest that RSV replication was inhibited in KK34. Identification of the STV11 gene STV11 was previously mapped to a 39.2-kb genomic interval containing seven annotated genes predicted to encode a sulfotransferase ( OsSOT1, LOC_Os11g30910), three hypothetical proteins (LOC_Os11g30899, LOC_Os11g30930, LOC_Os11g30950) and three retrotransposon proteins (LOC_Os11g30920, LOC_Os11g30940, LOC_Os11g30960), respectively [8] . Sequence analysis among KK34, Kos and Nipponbare (NIP) showed that each of the predicted genes carries one or more nucleotide substitutions, deletion or insertions, causing either amino acid (AA) substitutions, frame shift or pre-termination of the encoded gene products ( Supplementary Fig. 2 ). Real-time reverse transcriptase–PCR (RT–PCR) analysis showed that only OsSOT1 was obviously expressed in seedling leaves of Kos and KK34 ( Supplementary Fig. 3 ), thus OsSOT1 was selected as the candidate for STV11 . Sequence comparison of OsSOT1 revealed two non-synonymous nucleotide polymorphisms between KK34 and Kos, causing an AA substitution (T214S) and deletion of two alanine residues (AA224-225) in KK34, respectively ( Fig. 2a ). Moreover, sequence analysis of OsSOT1 in 24 varieties revealed that all thirteen RSV-resistant accessions have identical sequence to KK34, whereas all 11 RSV-susceptible accessions have the same sequence as Kos ( Fig. 2a ). The correlation between OsSOT1 sequence and RSV resistance strongly suggests that the KK34 allele is required for resistance to RSV. The Kos and KK34 alleles were thus designated STV11-S and STV11-R , respectively. In support of this, overexpression of S TV11-R, but not STV11-S, significantly inhibited RSV replication in leaf sheath protoplasts of the susceptible variety NIP ( Supplementary Fig. 4 ). Moreover, the overexpression of S TV11-R , but not STV11-S, conferred RSV resistance in susceptible N. benthamiana plants ( Supplementary Fig. 5 ). To further validate this result, we introduced a genomic fragment containing STV11-R coding sequence driven by its endogenous promoter or STV11 -R CDS driven by the maize ubiquitin-1 promoter into NIP. Notably, the transcript levels of both transgenes were induced by RSV infection ( Supplementary Fig. 6 ). All transgenic lines displayed significantly higher resistance to RSV, compared with the control ( Fig. 2b–g ). Together, these results support the notion that OsSOT1 corresponds to STV11 . 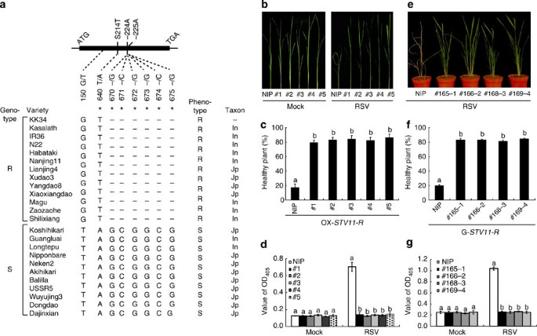Figure 2:STV11haplotypes and complementation tests. (a)STV11haplotypes identified in 24 rice varieties. AA changes are shown above the closed bar. *indicates non-synonymous polymorphisms. In,indica; Jp,japonica. (b–g) Acquired RSV resistance of transgenic lines overexpressingSTV11-R driven by the maizeUbiquitin-1promoter (b–d) or transformed with a genomic sequence ofSTV11-R(e–g). NIP, the susceptible wild type NIP. (c,f) Quantification of RSV resistance. (d,g) Measurement of RSV by ELISA assay. One-week-old plants were used for RSV infection. Photographing, resistant evaluation and ELISA were performed 30 (b–d) or 70 (e–g) d.p.i. Data are shown as means±s.e.m. (n=3). Different letters at the top of each column indicate a significant difference atP<0.01 (n=3) by the Student’st-test. Figure 2: STV11 haplotypes and complementation tests. ( a ) STV11 haplotypes identified in 24 rice varieties. AA changes are shown above the closed bar. *indicates non-synonymous polymorphisms. In, indica ; Jp, japonica . ( b – g ) Acquired RSV resistance of transgenic lines overexpressing STV11 -R driven by the maize Ubiquitin-1 promoter ( b – d ) or transformed with a genomic sequence of STV11-R ( e – g ). NIP, the susceptible wild type NIP. ( c , f ) Quantification of RSV resistance. ( d , g ) Measurement of RSV by ELISA assay. One-week-old plants were used for RSV infection. Photographing, resistant evaluation and ELISA were performed 30 ( b – d ) or 70 ( e – g ) d.p.i. Data are shown as means±s.e.m. ( n =3). Different letters at the top of each column indicate a significant difference at P <0.01 ( n =3) by the Student’s t -test. Full size image Expression, location and possible interaction studies of OsOST1 Real-time RT–PCR analysis showed that OsSOT1 was expressed in all tissues examined, with higher level at the seedling stage ( Supplementary Fig. 7a ). Furthermore, the expression of OsSOT1 was obviously induced by RSV infection ( Supplementary Fig. 7b ). To determine the subcellular location of OsSOT1 and whether there is translocation in response to inoculation with RSV, the STV11-R CDS was fused with the coding sequence of green fluorescent protein (GFP) gene under control of the CaMV 35S promoter and was co-expressed with various subcellular markers targeted to Golgi, endoplasmic reticulum (ER), mitochondria, cytoplasm or peroxisome in rice leaf protoplasts. Consistent with previously reported localization of some members of the sulfotransferases [11] , OsSOT1-GFP was co-localized with the ER maker mCherry–HDEL, the cis -Golgi marker GmMan1–mCherry and the trans -Golgi marker ST–mCherry ( Supplementary Fig. 8 ). No translocation of OsSOT1-GFP in the presence of RSV was observed ( Supplementary Fig. 8 ). To investigate whether OsSOT1 could directly interact with the RSV-encoded proteins to trigger a viral defense response, we examined possible interaction of OsSOT1 with each of the seven RSV-encoded proteins using the yeast two-hybrid assay. The results showed that OsSOT1 encoded by neither STV11-R nor STV11-S interacted with any of the RSV-encoded proteins ( Supplementary Fig. 9 ). OsSOT1 catalyses the conversion of SA into SSA SA is known to be involved in resistance to certain viruses [12] , [13] , [14] . A previous study showed that sulfotransferase encoded by AtSOT12 can sulphonate SA into SSA [15] , we thus conducted an in vitro enzymatic assay to test whether OsSOT1 is capable of sulphonating SA into SSA. We found that OsSOT1 encoded by STV11-R was indeed able to sulphonate SA into SSA, whereas OsSOT1 encoded by STV11-S could not ( Fig. 3a ). Computational homology modelling suggests that the AA residues varying between the OsSOT1s encoded by STV11-R and STV11-S are close to the sulphion-binding site of OsSOT1 ( Supplementary Fig. 10 ), indicating that these residues are functionally required for the sulfotransferase activity. Moreover, consistent with the previous observation that overexpression of AtSOT12 induced an increase in SA levels after pathogen infection [15] , we found that after infection by RSV, SA level in KK34 and transgenic plants expressing STV11-R were much higher than that in Kos and NIP ( Fig. 3b and Supplementary Fig. 11a ). These observations suggest that SSA may serve as a signal to trigger SA biosynthesis. In support of this notion, we found that expression of two SA biosynthesis related genes encoding phenylalanine ammonia-lyase and isochorismate synthase [16] was more significantly upregulated in KK34 than in Kos during RSV infection ( Supplementary Fig. 11b,c ). Together, these results suggest that the increased SA levels in KK34 and STV11-R transgenic lines may underlie the viral resistance. 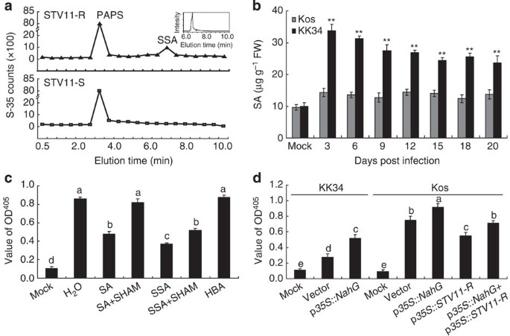Figure 3: Effect ofSTV11-Ron RSV resistance. (a) Sulfotransferase activities of STV11-R and STV11-S. The insert shows HPLC detection of the SSA standard. (b) SA contents in KK34 and Kos following RSV infection. Mock, the 1-week-old rice plants were not infected with RSV. Data are shown as means±s.e.m. (n=3), **indicates significant difference between Kos and KK34 at same time point atP<0.01 by the Student’st-test. (c) RSV replication is inhibited by SA or SSA in Kos protoplasts. Data are shown as means±s.e.m. (n=3). Different letters at the top of each column indicate a significant difference atP<0.05 (n=3) by the Student’st-test. (d) Increased RSV replication in KK34 protoplasts expressing the bacterial salicylate hydroxylase gene (NahG) and co-expression ofNahGreduces inhibition of RSV replication bySTV11-Rin Kos protoplasts. The protoplasts were collected at 16 h after infection of RSV. Mock (m), the protoplasts were not infected with RSV. Data are shown as means±s.e.m. (n=3). Different letters at the top of each column indicate a significant difference atP<0.05 (n=3) by the Student’st-test. Figure 3: Effect of STV11-R on RSV resistance. ( a ) Sulfotransferase activities of STV11-R and STV11-S. The insert shows HPLC detection of the SSA standard. ( b ) SA contents in KK34 and Kos following RSV infection. Mock, the 1-week-old rice plants were not infected with RSV. Data are shown as means±s.e.m. ( n =3), **indicates significant difference between Kos and KK34 at same time point at P <0.01 by the Student’s t -test. ( c ) RSV replication is inhibited by SA or SSA in Kos protoplasts. Data are shown as means±s.e.m. ( n =3). Different letters at the top of each column indicate a significant difference at P <0.05 ( n =3) by the Student’s t -test. ( d ) Increased RSV replication in KK34 protoplasts expressing the bacterial salicylate hydroxylase gene ( NahG ) and co-expression of NahG reduces inhibition of RSV replication by STV11-R in Kos protoplasts. The protoplasts were collected at 16 h after infection of RSV. Mock (m), the protoplasts were not infected with RSV. Data are shown as means±s.e.m. ( n =3). Different letters at the top of each column indicate a significant difference at P <0.05 ( n =3) by the Student’s t -test. Full size image To further investigate whether SA or SSA are functionally required to trigger RSV resistance, we compared the effects of SA and SSA on RSV replication in Kos protoplasts. We found that both SA and SSA significantly inhibited replication of RSV, with the latter being more effective ( Fig. 3c ). In contrast, an inactive isomer of SA, 3-hydroxybenzoic acid, could not block RSV replication ( Fig. 3c ). In addition, salicylhydroxamic acid (SHAM), a mitochondrial alternative oxidase inhibitor antagonizing SA-induced viral resistance [17] , fully blocked the inhibition of RSV replication by SA but it could only partially antagonize SSA treatment ( Fig. 3c ). The inhibition of RSV replication by SA and its alleviation by SHAM were also observed in N. benthamiana ( Supplementary Fig. 12 ). Moreover, reducing SA content in KK34 and Kos by heterologous expression of the bacterial salicylate hydroxylase gene ( NahG ) [18] resulted in increased replication of RSV ( Fig. 3d ). Further, the suppression of RSV replication by STV11-R was significantly attenuated in the presence of NahG in rice protoplasts and N. benthamiana plants ( Fig. 3d and Supplementary Fig. 5 ). Taken together, these data suggest that both SA and SSA can trigger a defense response against RSV in rice and N. benthamiana . Distribution pattern of STV11-R and STV11-S To trace the evolutionary origin and distribution patterns of STV11 , we sequenced the genomic sequence of OsSOT1 orthologs from 30 accessions of Oryza rufipogon , the progenitor of the cultivated rice in Asia [19] , [20] , [21] , [22] , [23] , and 271 varieties representing various periods of breeding history and geographic locations ( Fig. 4a ; Supplementary Data 1 ). A total of seven STV11 haplotypes were identified in Oryza rufipogon , but just three of them ( STV11-R , STV11-R′ and STV11-S ) were found in the analysed cultivars ( Fig. 4b ; Supplementary Data 1 and Supplementary Table 1 ). Only one non-synonymous polymorphism at AA 54 (A54V) was found between STV11-R and STV11-R′ . All tested varieties harbouring STV11-R′ showed high RSV resistance as KK34 ( Supplementary Table 2 , R =0.95, P =2.2 × 10 −16 ), indicating that STV11-R′ is functionally equivalent to STV11-R . Interestingly, the majority of Chinese O. rufipogon (9/11) carries STV11-S , whereas most of the South or Southeast O. rufipogon (14/19) carries either STV11-R or STV11-R′ ( Supplementary Table 1 ), suggesting that the STV11-R/R′ and STV11-S alleles already pre-existed in different geographic populations of O. rufipogon . Further, sequence analysis revealed that the majority of indica cultivars (85.03%, 125/147) carries either the STV11-R or the STV11-R′ resistance alleles. On the contrary, the majority of japonica accessions (77.42%, 96/124) have the susceptible STV11-S allele. These results provide a molecular explanation for the differential resistance of indica and japonica varieties to RSV and provide further support for the proposition that indica and japonica cultivars are derived from distinct geographic gene pools of a common wild ancestor [19] , [20] , [21] , [22] , [23] . 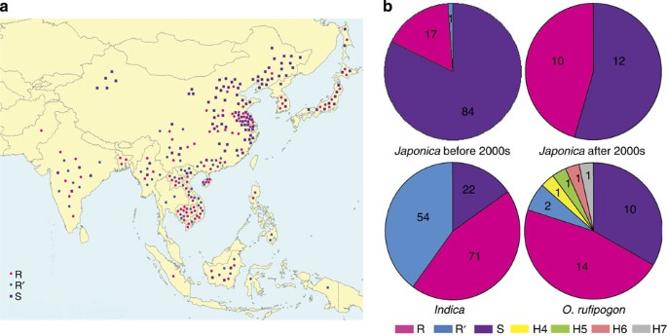Figure 4: Analysis of natural variation at theSTV11locus in rice cultivars andO. rufipogon. (a) Geographical origin of rice landraces and cultivars used in this analysis. (b) Distribution ofSTV11-RandSTV11-Sinjaponica,indicaandO.rufipogon. Figure 4: Analysis of natural variation at the STV11 locus in rice cultivars and O. rufipogon . ( a ) Geographical origin of rice landraces and cultivars used in this analysis. ( b ) Distribution of STV11-R and STV11-S in japonica , indica and O . rufipogon . Full size image STV11-R confers durable resistance to RSV Previous breeding programs to develop RSV resistance rice have mostly used the Pakistan indica cultivar Modan or the Japanese upland rice variety Kanto 72 (URK 72) as the resistance donor parent, which carry the Stvb-i or Stvb RSV resistance allele, respectively [5] , [24] , [25] . Previous mapping and allelic test suggested that both Stvb-i and Stvb are either tightly linked to or allelic with STV11 (refs 5 , 8 , 25 ). Intriguingly, our sequence analysis showed that Modan and Kanto 72, as well as their RSV-resistant offspring cultivars sequenced in this study all harbour the STV11-R allele ( Supplementary Table 3 ), providing further support for their allelism. Notably, the percentage of japonica cultivars carrying the STV11-R allele has increased from 16.67 to 45.45% since 2000s ( Fig. 4b ). These observations suggest that the STV11-R allele has been increasingly introgressed into more japonica cultivars from indica varieties during recent breeding programs to combat RSV. Strikingly, all STV11-R carrying varieties released since 1960s still retain effective resistance against RSV nowadays ( http://www.knowledgebank.irri.org/ ), suggesting that STV11-R confers durable resistance to RSV. In this study, we show that STV11, which confers durable resistance to RSV, encodes a sulfotransferase catalysing the conversion of SA into SSA, leading to increased SA accumulation in the RSV-infected plants and inhibition of viral replication. We also show that the resistant STV11-R and susceptible STV11-S alleles were predifferentiated in different geographic populations of the wild rice, Oryza rufipogon , and have remained prevalent in cultivated indica and japonica rice varieties, respectively. Our data provide a molecular explanation for the differential resistance of indica and japonica varieties to RSV. SA is known to be involved in resistance to kinds of biotic stress [12] , [13] , [14] , and it can be chemically modified in several ways, including glucosylation, methylation and AA conjugation. Most modifications render SA inactive, while at the same time they allow fine tuning of its accumulation, function and/or mobility [26] . For example, methylation inactivates SA while increasing its membrane permeability, as well as its volatility, thus allowing more effective long distance transport of this defense signal [27] . Glucosylation allows vacuolar storage of relatively large quantities of SA due to reduced toxicity [28] . In the present study, we demonstrated that STV11 encodes a sulfotransferase catalysing the conversion of SA into SSA and that SSA is more effective than SA in conferring RSV resistance and inhibition of viral replication. Notably, our data suggest that SSA may also serve as a signal to trigger increased biosynthesis of SA through a positive feedback mechanism after RSV infection. Similarly, it has been reported that sulphonation or sulphoconjugation can activate some hormonal substrates, such as pregnenolone and minoxidil [29] , [30] . On the contrary, sulphonation of hydroxyjasmonate by AtSOT15 was shown to play a role in JA inactivation in plants [31] . Thus, sulfotransferases can either positively or negatively regulate a biological process. Our sequence analysis also provided supporting evidence for the allelism of STV11-R with Stvb-i and Stvb , two previously reported RSV resistance genes used in breeding of RSV-resistant japonica varieties [5] , [24] , [25] . However, previous efforts to breed RSV-resistant rice varieties have been both time consuming and ineffective due to the lack of usable molecular markers tightly linked with the RSV resistance genes. We noted that all the japonica rice cultivars in Northeast China, the biggest japonica rice production region still carry the susceptible allele STV11-S , and the damage caused by RSV in this region is becoming increasingly severe recently [32] . The cloning of STV11 now should facilitate more effective breeding of RSV-resistant rice varieties through molecular marker-assisted selection and greatly aid in RSV management in the area. In addition to rice, RSV also can harm other graminaceous and nongraminaceous plant species, including the major staple crops wheat, maize and barley ( http://www.knowledgebank.irri.org/ ) [33] , [34] . Outbreaks of RSV in these species could constitute a major threat to global food production. Our study showed that heterologous transfer of rice STV11 into N. benthamiana plants could effectively block RSV replication, suggesting that STV11 is not only useful in breeding or genetic engineering RSV-resistant rice, but also possibly other crops, such as maize and wheat. Plant materials and growth conditions KK34 is a near isogenic line carrying STV11 from KAS in the genetic background of the susceptible japonica cultivar Koshihikari (Kos) [8] . Rice germplasms used in this work were obtained from the Chinese Crop Germplasm Resources Center (Beijing, China), the China National Rice Research Institute (Hangzhou, China), the Crop Germplasm Bank of Jiangsu Academy of Agricultural Sciences (Nanjing, China) and the Crop Germplasm Bank of Guangxi Academy of Agricultural Sciences (Nanning, China). Rice plants were grown in a greenhouse at 25–27 °C. N. benthamiana plants were grown in a growth chamber set at 25 °C and16 h light/8 h darkness conditions. Sequencing and homology modelling The DNA sequence in the STV11 region was downloaded from the genome database of Oryza sativa subsp. japonica cv. NIP ( http://www.ncbi.nlm.nih.gov ) and used for gene prediction. Gene models were obtained from GRAMENE ( http://www.gramene.org ). Seven predicted genes in the fine mapped 39.2-kb region were sequenced for Kos and KK34. The primers were listed in Supplementary Table 4 . The structure of Arabidopsis sulfotransferases was used as the template for constructing the structure model of STV11. Sequences were aligned by the Align 2D structure alignment programme (Homology module, InsightII; Accelrys). Structures were automatically built by the MODELER module of InsightII. Vector construction and plant transformation For genetic complementation, a 1.2-kb DNA fragment containing the entire STV11-R coding region was PCR amplified using gene-specific primers UBI- STV11-R ( Supplementary Table 4 ) from KK34 seedling genomic DNA, and inserted into Kpn I and BamH I-digested binary vector pCUBI1390. The transgene was driven by the maize ubiquitin promoter. A 7,867-bp STV11-R genomic DNA fragment including 2,706 bp of upstream sequence, the full-length STV11-R coding region and 835 bp of downstream sequence was amplified from the KK34 genomic DNA and cloned into the EcoR I site of the binary vector pCAMBIA1305.1 using In-Fusion Advantage PCR Cloning Kits (Clontech) to generate the plasmid G- STV11-R . The complementation construct was transformed into the rice NIP variety, using an Agrobacterium -mediated method. Plants regenerated from hygromycin-resistant calli (T 0 plants) were grown in padding field in Nanjing Agricultural University, and T 1 seeds were obtained after self-pollination. T 2 seedlings were used for RSV resistance evaluation. To construct the transforming vector p 35S - STV11-R ( S ) for N. benthamiana plants and protoplasts, the STV11 coding sequence was PCR amplified from KK34 (Kos) cDNA and cloned into Kpn I and BamH I-digested binary vector p2300S, resulting in the plasmid p 35S - STV11-R ( S ) (The transgene was driven by the CaMV 35S promoter). To investigate the cellular localization of STV11, the OsSOT1 coding sequence was PCR amplified from KK34 cDNA was fused in frame with GFP and inserted between the CaMV 35S promoter and the NOS terminator in the pAN580 vector (The primer p OsSOT1 -GFP was showed in Supplementary Table 4 ). To obtain the purified STV11 recombinant protein in vitro , the KK34 and Kos STV11 cDNA were amplified using the primer GEX- STV11 ( Supplementary Table 4 ) and cloned into the pGEX-4T-2 expression vector (GE Life Science). The recombinant proteins were purified using the GSTrap FF columns and HiTrap Benzamidine FF (GE Healthcare). Inoculations of RSV in rice and N. benthamiana plants Laodelphax striatellus were maintained on rice seedlings in an insect-rearing room. To obtain viruliferous insects, nymphs were reared on virus-infected rice plants for 2 days, and insects were maintained up to the adult stage with occasional replacement of healthy rice seedlings. Thirty germinated seeds of each line were sown in plastic dishes filled with soil; the weak seedlings were eliminated at the one-leaf stage, and 25 healthy seedlings of each line were kept for inoculation. When the seedlings were at the one-and-half-leaf stage, the rice plants were inoculated by exposure to five to seven viruliferous SBPHs per plant for 2 days. During inoculation, the SBPHs in each dish were disturbed with a small soft brush every day to avoid aggregation. Two days later, all SBPH nymphs were killed with pesticide and seedlings were transferred to a greenhouse, where they grew for about a month until symptom examination. The reaction to RSV was evaluated by calculating the proportion of healthy plants (the percentage of healthy plants in a given plot). Plants with yellow and white stripe disease lesions and more severe symptoms were considered susceptible plants. In contrast, plants without typical disease lesions or those that exhibited slight symptoms or disappeared were considered resistant plants. RSV infectivity trials on N. benthamiana plants were performed according to Xu and Zhou [35] with some modifications. In brief, N. benthamiana plants were carried out by rub-inoculating leaves with crude extracts from RSV-infected O. sativa leaves ground in a phosphate buffer (0.2 M). The preantepenultimate leaves of 4-week-old N. benthamiana plants were infiltrated with Agrobacterium tumefaciens (strainGV3101) harbouring vector p2300S, NahG overexpression consturct [36] , p 35S - STV11-S , p 35S-STV11-R or p 35S-STV11-R plus the NahG overexpression construct using needleless syringes 30 h before RSV infection. The chlorosis and yellowing symptoms in the systemic leaf were observed at 15 d.p.i. For SA and SA plus SHAM treatment, 3-week-old N. benthamiana plants were sprayed with solutions of 1 mM SA or 1 mM SA plus 2 mM SHAM for 5 days before RSV infection. Evaluation of SBPH resistance Three methods were used to evaluate SBPH resistance. (1) Modified seedbox screening test. At the 1.5- to 2.0-leaf stage, the seedlings were infested with second to third instar SBPH nymphs at 15 insects per seedling. The mortality rate of plants on each variety was calculated when above 90% of Wuyujing 3 seedlings were dead; (2) Antixenosis test. At the 1.5- to 2.0-leaf stage, seedlings were transferred into cages covered with nylon net and infested with 2nd to 3rd instar BPH nymphs at five insects per seedling. The average number of insects on each entry at 4 d.p.i. was regarded as the value of antixenosis; (3) Antibiosis test. At the 1.5- to 2.0-leaf stage, seedlings were infested with 1- to 2-instar SBPH nymphs at 20 insects per seedling. At 1, 3, 5 and 7 days after infestation, the survival rate of insects on each variety was calculated, respectively. Details of the procedures have been described previously [37] . Virus and protoplast isolation and ELISA analysis RSV was isolated and purified from rice plants infected with RSV as described [38] with some modifications. Briefly, about 100 g of leaves freshly collected or stored below −20 °C, were blended in 400 ml phosphate buffer (0.1 M, pH 7.5) containing 0.1% 2-Mercaptoethanol, 1% Triton X-100 and 0.01 M EDTA. The homogenate was squeezed through two layers of gauze, mixed with 40 ml chloroform and stirred for 10 min. After clarification by centrifugation for 20 min at 5,000 g , the supernatant was adjusted to 6% polyethylene glycol 6,000 and 0.1 M NaCl in an ice-bath for 4 h and then kept at 4 °C overnight. The precipitate was collected by centrifugation for 20 min at 5,000 g and the pellets were dissolved in 0.01 M phosphate buffer pH 7.5. After centrifugation for 10 min at 5,000 g , the supernatant was centrifuged for 2 h at 100,000 g . The pellets were again dissolved in the 0.01 M phosphate buffer pH 7.5 and the virus particles were pelleted by centrifugation for 2 h at 100,000 g in 20% glycerol. The virus particle pellets were removed with a syringe, either separately or in combination and were dissolved in 0.01 M phosphate buffer pH 7.5. Purified virus particles were characterized by 12% SDS-polyacrylamide gel electrophoresis, and the virus concentration was determined using the Bradford assay with bovine serum albumin as a standard. Purified particles were stored at −70 °C. Protoplast isolation from rice and transfection were performed as described [39] , [40] with some modifications. The protoplasts were stored on ice for 30 min before transfection. The protoplasts were counted in a hemocytometer and prepared at a density of 5 × l0 6 protoplasts per ml. The protoplasts were collected and resuspended in the same volume of protoplast suspension medium (0.4 M mannitol, 20 mM CaCl 2 2H 2 O, and 5 mM Mes-KOH, pH 5.7). Then, 200 μl of protoplast solutions was mixed with 100 μg salmon sperm carrier DNA, 1 μg RSV particles and 10 μg plasmid. Next, 220 μl of polyethylene glycol-CHS solution (0.4 M mannitol, 0.1 M CaCl 2 2H 2 O, and 40% polyethylene glycol 4,000) was added to the protoplast-plasmid mixture and incubated for 20 min at room temperature. Then, 1 ml of W5 buffer was added slowly to the mixture and the sample was washed with W5 buffer for three times. The transfected protoplasts were resuspended in 1 ml of W5 buffer and incubated in the dark at 28 °C. The infected protoplasts were collected at different times after infection and stored at −20 °C. The replication of RSV in the transfected protoplasts and the accumulation of RSV in newly emerged leaves of infected/mock plants were measured by indirect enzyme-linked immunosorbent assay (ELISA). In the ELISA system, the anti-mouse primary antibody for RSV and the alkaline phosphatase-conjugated secondary antibody were obtained from Dr Xueping Zhou (Zhejiang University, Hangzhou, China) and purchased from Sigma (St Louis, MO, USA), respectively. The antibody was used at a 1:3,000 dilution. Subcellular localization The expression construct was transfected into rice protoplasts according to the protocols as described [39] , [40] with some modifications. Briefly, 10 μg of plasmid DNA were mixed with 200 μl protoplasts of each sample (about 1 × 10 6 cells). Freshly prepared polyethylene glycol solution (220 μl; 40% (w/v)) polyethylene glycol 4,000, 0.2 M mannitol and 0.1 M CaCl 2 ) were added, and the mixture was incubated at room temperature for 20 min in the dark. After incubation, 1 ml W5 solution was added to the samples slowly. The resulting solution was mixed well by gently inverting the tube, and the protoplasts were pelleted by centrifugation at 1,500 r.p.m. for 3 min. The protoplasts were resuspended gently in 1 ml W5 solution. Finally, the protoplasts were transferred into multi-well plates and cultured under light or darkness at room temperature for 16 h. The well-established fluorescent protein markers used were mCherry–HDEL for the ER [41] , ST–mCherry for the trans -Golgi [42] and GmMan1–mCherry for the cis -Golgi [41] . The samples were observed with a confocal laser scanning microscope (Leica TCS SP5). RNA isolation and quantitative real-time RT–PCR analysis Total RNA was isolated from rice seedlings using the RNAprep Pure Plant Kit (Tiangen) according to the manufacturer’s instructions. Quantitative RT–PCRs were performed by a SYBR Premix Ex Taq RT–PCR Kit (Takara) following the manufacturer’s instructions with the primers listed in Supplementary Table 4 . Relative transcript levels were calculated by formula 2 (Ubiquitin Ct−Target Ct) following the method [43] with the OsRubq1 as an internal control. Sulphotransferase activity assay The sulphotransferase activity of STV11 protein was measured by using radio-HPLC (high-performance liquid chromatography) method. [ 35 S]-phosphoadenosine phosphosulphate (PAPS, PerkinElmer Life and Analytical Sciences, http://www.perkinelmer.com ) was used as the sulphate donor to maximize the detection sensitivity. The detailed procedure was performed as described [15] with some modifications. In brief, the reaction in a mixture (100 μl) containing 10 μl of [ 35 S]-PAPS, 10 μg of purified STV11 protein, 1 mM substrate (SA) and 50 mM MES buffer, pH 5.5 was allowed to proceed for 30 min at 30 °C and then stopped by adding three volumes of cold methanol and incubated at −80 °C for 2 h. After centrifuging at 12,000 g for 10 min to precipitate the proteins, the supernatant was transferred to a new tube and dried under speed vacuum. The enzymatic reaction remnant was dissolved in ice-cold 50% methanol and subjected to HPLC fractionation (Agilent 1,200 Series, Agilent Technologies ZORBAX Eclipse XDB-C18 column, mobile phase: methanol with 1% acetic acid, 25% methanol within 20 min). Then, 40 fractions (one fraction per 30 s) were collected using the BS-160A fraction collector (Shanghai, China). The radioactivity in each fraction was measured by liquid scintillation counting (Beckman, LS 6500). SA measurement SA was extracted from 0.1 g (fresh weight) of leaf tissue and quantified with a biosensor strain Acinetobacter species, ADPWH_ lux , as described [44] , [45] , [46] with some modifications. Briefly, samples were ground three times at 1,500 strokes per min for 30 s in a Mixer Mills MM400 (VERDER RETSCH) while refreezing in liquid nitrogen each time. Then, samples were left at room temperature for 5 min, and 2.5 μl acetate buffer (0.1 M, pH 5.6) per milligram tissue was added. Samples were then mixed for 1 min at 1,000 strokes per min and centrifuged for 15 min at 13,000 g . The supernatant was stored on ice for free SA measurement. Overnight cultured Acinetobacter sp. ADPWH_ lux were diluted with lysogeny broth (1:20) and grown for ~3 h at 200 r.p.m. to an OD 600 of 0.4–0.5 at 37 °C. Crude (20 μl) extract was added to 60 μl LB in a black 96-well black cell culture plate at room temperature. Using a multipipet, 50 μl of biosensor culture was added to each well and mixed by pipet action. The plate was incubated at 37 °C for 1 h without shaking before luminescence was read using a SpectraMax M3 Multi-Mode Microplate Reader (Molecular Devices, Sunnyvale, California). Each sample was measured in triplicate. The NIP NahG transgenic line that has no detectable SA level [36] was used for the standard curve construction. How to cite this article: Wang, Q. et al. STV11 encodes a sulphotransferase and confers durable resistance to rice stripe virus. Nat. Commun. 5:4768 doi: 10.1038/ncomms5768 (2014).